DNase II-dependent DNA digestion is required for DNA sensing by TLR9 DNase II digests DNA in endolysosomes. In the absence of DNase II, undigested DNA activates cytoplasmic DNA-sensing pathways. Little is known, however, about the role of DNase II in endolysosomal DNA sensing by TLR9. Here we show that DNase II is required for TLR9. We test two types of TLR9 ligands, CpG-A and CpG-B, and show that only CpG-A response is impaired in DNase II-deficient dendritic cells (DCs). Enzymatically inactive DNase II mutants cannot rescue CpG-A responses. DNase II cleaves CpG-A from 20-mer to 11-12-mer. The 3′11-mer CpG-A fragment activates DNase II-deficient DCs. CpG-A shows higher co-localization with LAMP-2 + lysosomes than CpG-B and induces DNase II localization in LAMP-2 + lysosomes. Moreover, we demonstrate that DNase II is required for TLR9 activation by bacterial genomic DNA. Taken together, these results demonstrate that TLR9 responds to DNA fragments generated by DNase II. The innate immune system is the first line of defence against infection. Pathogen sensors recognize a wide range of microbial products and activate inflammatory responses. DNA has emerged as one of the major activators of innate immune responses [1] . The best-studied DNA sensor is Toll-like receptor 9 (TLR9), which is localized in endolysosomes and senses endocytosed single-stranded DNA (ssDNA) containing CpG dinucleotide [2] . Three distinct types of oligodeoxynucleotides (ODNs) have been described [3] . CpG-A induces large amounts of type I interferon (IFN) in plasmacytoid DCs, whereas CpG-B strongly activates B cells. A third class of CpG ODN, CpG-C, combines the immune effects of CpG-A and CpG-B ODNs [4] . CpG-A and CpG-C, but not CpG-B, have the CpG-containing palindromic region and CpG-A forms nanoparticles in endolysosomes [5] . These properties are thought to be essential for IFN-α induction, but the underlying mechanisms have not been fully elucidated. Self/pathogen discrimination by TLR9 is error-prone and needs to be strengthened by compartmentalization of DNA sensing in endolysosomes, instead of on the cell surface. Although self-derived DNA is rapidly degraded by nucleases, microbial nucleic acids are resistant to degradation, because they are encased in bacterial cell walls or viral coat proteins. Thus, microbial DNA, but not self-derived nucleic acids, reaches endolysosomes and stimulates TLRs [6] . In autoimmune diseases such as systemic lupus erythematosus (SLE) and psoriasis, self-DNA is complexed with autoantibodies or the cationic antimicrobial peptide LL37. These complexes are resistant to degradation, delivered into endosomal compartments by endocytosis and activate TLR9, leading to DC activation and production of inflammatory cytokines [7] , [8] , [9] . A role of DNA digestion in preventing autoimmunity is corroborated by studies on neutral DNase I in the circulation, acidic DNase II in lysosomes and cytoplasmic DNase III (also known as the 3′ repair exonuclease 1, Trex1). Loss-of-function mutations in DNase I predispose to SLE in humans and mice [10] , [11] . Dnase1 −/− mice show SLE-like diseases with anti-nuclear antibody production, such as the deposition of immune complexes in glomeruli and full-blown glomerulonephritis [11] . On the other hand, Dnase2a −/− mice show embryonic death due to anaemia as a consequence of constitutive production of IFN-β. Dnase2a −/− Ifnar1 −/− double-deficient mice are born normally but suffer from chronic polyarthritis, due to constitutive production of tumour necrosis factor-α (TNF-α) [12] . Mutations in DNase III cause Aicardi–Goutières syndrome, a type I IFN-associated autoimmune disease in humans [13] . Type I IFN production is induced by activating stimulator of type I IFN gene ( STING ), an essential signalling adaptor for cytoplasmc DNA sensors [14] . It is important to understand how DNA degradation influences DNA sensors. In this regard, it is of note that cytoplasmic DNA sensors rather than endosomal TLR9 are activated in Dnase2a −/− mice. IFN-β-dependent lethality and chronic arthritis are not found in mice lacking both DNase II and STING [15] . Even though endogenous DNA accumulates in lysosomes in Dnase2a −/− mice, TLR9 is not required for IFN-β production [16] . These results raise a question on TLR9 responses in Dnase 2a −/− immune cells. The present study focuses on TLR9 responses in Dnase2a −/− Ifnar1 −/− mice and shows an indispensable role of DNase II in TLR9 responses to CpG-A. CpG-A digestion by DNase is required for TLR9 responses. CpG-A fragments are generated by DNase II-dependent cleavage. The 11- and 12-mer fragments from 3′-end, but not 9- or 10-mer, activates DNase II-deficient DCs. Moreover, DNase II is required for TLR9 activation by bacterial genomic DNA. Taken together, TLR9 responds to DNA fragments generated by DNase II. CpG-A response is selectively impaired in Dnase2a −/− BM-cDCs To study the role of DNase II in DNA sensing by TLR9, the Dnase2a −/− Ifnar1 −/− mice were used. Although DNase II deficiency causes systemic inflammation, bone marrow-conventional DCs (BM-cDCs) did not show any alteration in terms of expression of cell surface markers such as CD11b and CD11c ( Fig. 1a ). Expression and proteolytic cleavage of TLR9 were not altered either ( Fig. 1b ). These cells were stimulated with the TLR9 ligands, CpG-A and CpG-B, or the TLR4 ligand lipid A as the control. The Dnase2a −/− Ifnar1 −/− BM-cDCs showed severely impaired production of IL-12p40 and regulated on activation, normal T cell expressed and secreted (CCL5, RANTES) in response to CpG-A ( Fig. 1c,d ). CpG-B responses were not altered at lower concentration. CpG-A and CpG-B did not activate Tlr9 −/− BM-cDCs ( Supplementary Fig. 1a ), confirming the specificity of the ligands used in the present study. Lipid A responses Dnase2a −/− Ifnar1 −/− BM-cDCs were not altered at all. Moreover, no alteration was found in IL-12p40 production in response to a TLR7 ligand RNA9.2 or a STING ligand 3′3′ cGAMP ( Supplementary Fig. 1b ). The 3′3′ cGAMP used in the present study was confirmed to be unable to stimulate Tmem173 −/− BM-cDCs ( Supplementary Fig. 1c ). BM-cDCs did not produce IL-12p40 in response to double-straned RNA (dsRNA) poly(I:C) or to the lipofectamine (LF)-complexed double-stranded DNA (dsDNA; interferon stimulatory DNA (ISD) or poly(dA:dT)) or dsRNA ( Supplementary Fig. 1b,c ). The STING pathway may preferentially induce type I IFN in BM-cDCs. 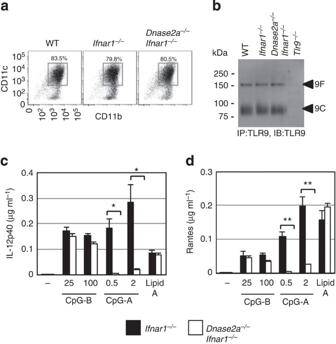Figure 1: Impaired CpG-A response inDnase2a−/−Ifnar1−/−BM-cDCs. (a) Dot plots showing expression of cell surface markers on BM-cDCs from WT,Ifnar1−/−andDnase2−/−Ifnar1−/−mice. (b) Immunoprecipitation and immunoblotting of TLR9 from WT,Ifnar1−/−andDnase2−/−Ifnar1−/−BM-cDCs are shown. Full-length TLR9 (9F) and the C-terminal fragment of cleaved TLR9 (9C) are indicated by arrowheads. BM-cDCs fromIfnar1−/−orDnase2−/−Ifnar1−/−mice were stimulated with indicated TLR ligands and production of IL-12 p40 (c) and RANTES (d) was evaluated by ELISA assay. Data representative of at least three independent trials are shown. Error bars indicate s.d. Statistical analyses were calculated using the Student’st-test (*P<0.05; **P<0.01). Figure 1: Impaired CpG-A response in Dnase2a −/− Ifnar1 −/− BM-cDCs. ( a ) Dot plots showing expression of cell surface markers on BM-cDCs from WT, Ifnar1 −/− and Dnase2 −/− Ifnar1 −/− mice. ( b ) Immunoprecipitation and immunoblotting of TLR9 from WT, Ifnar1 −/− and Dnase2 −/− Ifnar1 −/− BM-cDCs are shown. Full-length TLR9 (9F) and the C-terminal fragment of cleaved TLR9 (9C) are indicated by arrowheads. BM-cDCs from Ifnar1 −/− or Dnase2 −/− Ifnar1 −/− mice were stimulated with indicated TLR ligands and production of IL-12 p40 ( c ) and RANTES ( d ) was evaluated by ELISA assay. Data representative of at least three independent trials are shown. Error bars indicate s.d. Statistical analyses were calculated using the Student’s t -test (* P <0.05; ** P <0.01). Full size image CpG-A response is impaired in conditional Dnase2a −/− BM-pDCs CpG-A is known to robustly induce type I IFN in BM-plasmacytoid DCs (pDCs), and that type I IFN in turn strongly influences pDC responses [17] ; it is not appropriate to study BM-pDCs responses in the absence of type I IFN signalling. Therefore, instead of the Dnase2a −/− Ifnar1 −/− mice, the Dnase2a flox/flox Tie2-Cre mice were used. The expression level of DNase II messenger RNA in Dnase2a flox/flox Tie2-Cre BM-pDCs was reduced by 80%, while cell surface expressions of B220 and CD11c were not altered ( Supplementary Fig. 2 ). BM-pDCs were stimulated with CpG-A or CpG-B, and cytokine production was evaluated by enzyme-linked immunosorbent assay (ELISA). Production of IL-12 p40, RANTES, interleukin (IL)-6, TNF-α and IFN-α after stimulation with CpG-A was all significantly impaired in Dnase2a flox/flox Tie2-Cre BM-pDCs ( Fig. 2a–e ), but the CpG-B responses were not impaired. Partial impairment is probably due to residual expression of DNase II in Dnase2a flox/flox Tie2-Cre BM-pDCs ( Supplementary Fig. 2a ). These results suggest that CpG-A responses in BM-pDCs are dependent on DNase II. 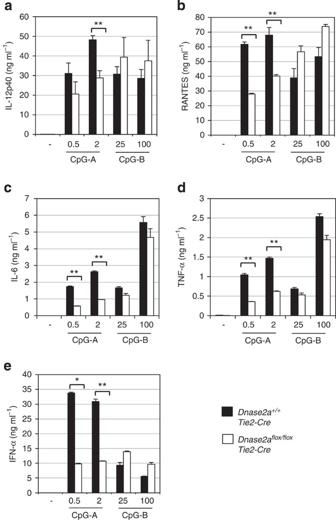Figure 2: Impaired CpG-A responses inDnase2aflox/floxTie2-CreBM-pDCs. (a–e) BM-pDCs were stimulated with CpG-A or CpG-B at the indicated concentrations. Production of IL-12 p40, RANTES, IL-6, TNF-α and IFN-α was determined by ELISA assay. Data representative of three independent trials are shown. Error bars indicate s.d. Statistical analyses were calculated using the Student’st-test (*P<0.05; **P<0.01). Figure 2: Impaired CpG-A responses in Dnase2a flox/flox Tie2-Cre BM-pDCs. ( a – e ) BM-pDCs were stimulated with CpG-A or CpG-B at the indicated concentrations. Production of IL-12 p40, RANTES, IL-6, TNF-α and IFN-α was determined by ELISA assay. Data representative of three independent trials are shown. Error bars indicate s.d. Statistical analyses were calculated using the Student’s t -test (* P <0.05; ** P <0.01). Full size image DNase activity is required for TLR9 responses to CpG-A To gain a mechanistic insight into the role of DNase II in CpG-A responses, the requirement for DNase activity was investigated. Histidine at the amino acid positions 115, 132 and 297 are indispensable for DNase activity in porcine DNase II [18] . Mouse DNase II mutants replacing H115 or H297 with alanine (H115A and H297A, respectively) were purified. H115A and H297A mutants showed slower migration than wild type (WT) DNase II in SDS–polyacrylamide gel electrophoresis (SDS–PAGE; Fig. 3a ). As suggested in the previous report [18] , these mutations may influence glycosylation of DNase II. The DNase activities of these mutants were evaluated by incubation with plasmid DNA. H297A DNase II failed to degrade DNA ( Fig. 3b ) and the H115A mutant showed only residual activity after 24 h. Next, stem cell-enriched BM cells from Dnase2a −/− Ifnar1 −/− mice were transduced with retrovirus vectors encoding WT, H115A or H297A DNase II tagged with green fluorescent protein (GFP). After transduction, BM cells were allowed to differentiate into BM-cDCs. All the DNase II constructs were comparably expressed, as examined by fluorescence-activated cell sorting (FACS) analyses ( Fig. 3c ). BM-cDCs were stimulated with CpG-A or CpG-B, and cytokine production was examined. CpG-A-dependent production of IL-12p40 and RANTES was rescued only by WT DNase II but not the mutants ( Fig. 3d ). In contrast, overexpression of DNase II did not alter CpG-B responses in Dnase2a −/− Ifnar1 −/− BM-cDCs. These results demonstrate that DNase II-dependent DNA degradation is indispensable for CpG-A sensing by TLR9. 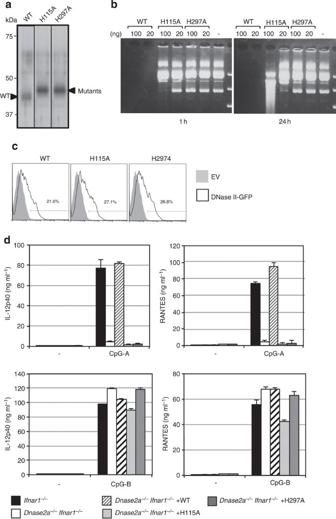Figure 3: Requirement for DNase activity in TLR9 responses to CpG-A. (a) WT DNase II and its mutants, H115A and H297A, were purified and analysed by SDS–PAGE and then silver staining. (b) Plasmid DNA was left untreated (−) or incubated with the indicated amounts of WT or mutant DNase II proteins for 1 or 24 h. DNA fragments were visualized by agarose gel electrophoresis. (c) Open histograms show comparable expression of WT, H115A and H297A DNase II-GFP inDnase2a−/−Ifnar1−/−BM-cDCs. Gray histograms show BM-cDCs expressing empty vector (EV). (d) BM-cDCs shown incwere stimulated with CpG-A or CpG-B. Production of IL-12p40 and RANTES was evaluated by ELISA assay. Data representative of three independent trials are shown. Error bars indicate s.d. Figure 3: Requirement for DNase activity in TLR9 responses to CpG-A. ( a ) WT DNase II and its mutants, H115A and H297A, were purified and analysed by SDS–PAGE and then silver staining. ( b ) Plasmid DNA was left untreated (−) or incubated with the indicated amounts of WT or mutant DNase II proteins for 1 or 24 h. DNA fragments were visualized by agarose gel electrophoresis. ( c ) Open histograms show comparable expression of WT, H115A and H297A DNase II-GFP in Dnase2a −/− Ifnar1 −/− BM-cDCs. Gray histograms show BM-cDCs expressing empty vector (EV). ( d ) BM-cDCs shown in c were stimulated with CpG-A or CpG-B. Production of IL-12p40 and RANTES was evaluated by ELISA assay. Data representative of three independent trials are shown. Error bars indicate s.d. Full size image Cleavage of CpG-A by DNase II is required for TLR9 response Requirement for DNase activity in CpG-A responses suggests direct cleavage of CpG-A by DNase II. To address this possibility, CpG-A was incubated with purified murine DNase II and DNA cleavage was evaluated by electrophoresis. A small but significant amount of cleaved fragment was detected by treatment with WT DNase II but not its mutants ( Fig. 4a ). All the nucleotides in CpG-B are phosphorothioated and thereby resistant to DNA cleavage. No cleavage was seen in CpG-B incubated with DNase II ( Fig. 4a ). CpG-A contains DNase-sensitive phosphodiester backbone in the central CpG-containing palindromic motif and the DNase-resistant phosphorothioated backbone at both ends ( Fig. 4b ). If the DNase-sensitive central portion is cleaved by DNase II, a fragment of about 10 bases would be generated. Truncated CpG-A fragments consisting of 9 to 13-mer at the 3′-end were synthesized ( Fig. 4b ). Comparing these truncated fragments with the cleaved CpG-A generated by DNase II digestion, the cleaved fragment appeared to be 11 or 12 bases in length ( Fig. 4c ). If cleavage of CpG-A by DNase II is required for TLR9 responses, truncated CpG-A fragments should be able to activate the Dnase2a −/− Ifnar1 −/− BM-cDCs. BM-cDCs were stimulated with each of the four ODNs: A5′09, A5′11, A3′09 and A3′11. Among them, the 11-mer from the 3′end (A3′11) was able to induce cytokine production in WT BM-cDCs but not in Tlr9 −/− BM-cDCs. The transfection reagent, LF, augmented A3′11 response, suggesting that the delivery of half-sized CpG-A to TLR9 is strengthened by LF. 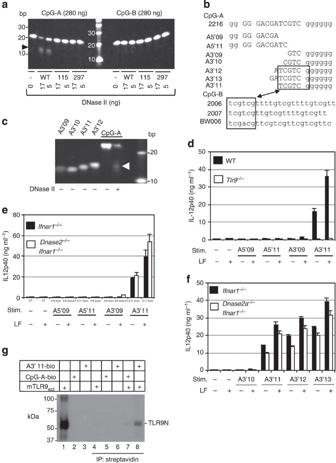Figure 4: The 3′ half of CpG-A is able to activate DNase II-deficient BM-cDCs. (a) CpG-A and CpG-B (280 ng each) were treated with increasing amounts (5, 17 ng) of WT or mutant DNase II for 24 h, and the cleaved fragments were visualized by TBE gel electrophoresis. The arrowhead indicates cleaved CpG-A. (b) The sequences of the CpG-A fragments synthesized for analyses. Lower case stands for the modification by phosphorothioated backbone. The sequences of CpG-B ODNs are also shown. Boxed CpG-B sequences represent the region similar to the boxed sequence in A3′11-13. (c) Uncleaved and cleaved CpG-A were compared with truncated CpG-A ODNs (A3′09-12) in TBE gel. The white arrowhead indicates cleaved CpG-A fragments. (d) BM-cDCs from WT orTlr9−/−mice were stimulated with truncated CpG-A fragments. IL-12p40 production was evaluated by ELISA assay. The results are represented by the average value with s.d. from triplicated wells. (e,f) BM-cDCs fromIfnar1−/−orDnase2a−/−Ifnar1−/−mice were stimulated as ind. (g) Biotinylated A3′11 or CpG-A (500 pmol each) was mixed with mouse TLR9 ectodomain (mTLR9ect) (~1 μg) for 1 h on ice and precipitated with streptavidin. Precipitated TLR9 ectodomain was subjected to immunoblotting for the N-terminal fragment of proteolytically cleaved TLR9 (TLR9N). Lane 1: the amount of mTLR9 ectodomain for interaction with biotinylated oligo DNA (~1 μg). Data representative of at least three independent trials are shown. Error bars in ELISA assay results indicate s.d. Figure 4: The 3′ half of CpG-A is able to activate DNase II-deficient BM-cDCs. ( a ) CpG-A and CpG-B (280 ng each) were treated with increasing amounts (5, 17 ng) of WT or mutant DNase II for 24 h, and the cleaved fragments were visualized by TBE gel electrophoresis. The arrowhead indicates cleaved CpG-A. ( b ) The sequences of the CpG-A fragments synthesized for analyses. Lower case stands for the modification by phosphorothioated backbone. The sequences of CpG-B ODNs are also shown. Boxed CpG-B sequences represent the region similar to the boxed sequence in A3′11-13. ( c ) Uncleaved and cleaved CpG-A were compared with truncated CpG-A ODNs (A3′09-12) in TBE gel. The white arrowhead indicates cleaved CpG-A fragments. ( d ) BM-cDCs from WT or Tlr9 −/− mice were stimulated with truncated CpG-A fragments. IL-12p40 production was evaluated by ELISA assay. The results are represented by the average value with s.d. from triplicated wells. ( e , f ) BM-cDCs from Ifnar1 −/− or Dnase2a −/− Ifnar1 −/− mice were stimulated as in d . ( g ) Biotinylated A3′11 or CpG-A (500 pmol each) was mixed with mouse TLR9 ectodomain (mTLR9 ect ) (~1 μg) for 1 h on ice and precipitated with streptavidin. Precipitated TLR9 ectodomain was subjected to immunoblotting for the N-terminal fragment of proteolytically cleaved TLR9 (TLR9N). Lane 1: the amount of mTLR9 ectodomain for interaction with biotinylated oligo DNA (~1 μg). Data representative of at least three independent trials are shown. Error bars in ELISA assay results indicate s.d. Full size image Very importantly, A3′11-mer was able to induce IL-12p40 production from Dnase2a −/− Ifnar1 −/− BM-cDCs as much as from Ifnar1 −/− BM-cDCs ( Fig. 4e ). To further study the requirement for activation of DNase II-deficient BM-cDCs, A3′10, A3′12 and A3′13 were also studied. Only A3′10 failed to stimulate Dnase2a −/− Ifnar1 −/− BM-cDCs ( Fig. 4f ). Interestingly, all the active CpG-A 3′ODNs share the CpG-containing sequence 5′- TCGTCg -3′, which is known to activate TLR9 (ref. 2 ) and found also in CpG-B ( Fig. 4b ). To gain a mechanistic insight underlying TLR9 activation by A3′11, TLR9 interaction with CpG-A or A3′11 was studied. Biotinylated CpG-A or A3′11 was mixed with the purified ectodomain of mouse TLR9. The ODNs were precipitated by streptavidin and co-precipitation of the TLR9 ectodomain was detected by immunoblotting. The TLR9 ectodomain are known to be cleaved into two fragments TLR9N and TLR9C, which are associated with each other [19] . The amino-terminal fragment was detected by immunoblotting. A larger amount of TLR9 fragments were precipitated with A3′11 than full-length CpG-A ( Fig. 4g , compare lane 7 with 8), suggesting that CpG-A poorly binds to TLR9 ectodomain. These results strongly suggest that TLR9 binds to the cleaved CpG-A fragment. DNase II traffics into lysosomes on CpG-A stimulation If CpG-A is cleaved into CpG-B-like fragment by DNase II, it raises a question why only CpG-A strongly induces IFN-α. CpG-A and CpG-B are distinct from each other in their subcellular distributions and the distribution of CpG-A has been shown to have strong impact on TLR9 responses [20] , [21] . CpG-A activates TLR9 in LAMP-2 + lysosomes or lysosome-related organelles [22] . The present study shows that DNase II is selectively required for CpG-A responses, suggesting that DNase II is localized also in lysosomes or lysosome-related organelles. To study the subcellular distribution of DNase II, anti-DNase II monoclonal antibody (mAb) was established. The specificity of the mAb was verified by immunoprecipitation. DNase II was precipitated from WT, Tlr9 −/− and Ifnar1 −/− , but not from Dnase2a −/− Ifnar1 −/− BM-cDCs ( Supplementary Fig. 4a ). As reported previously [23] , the apparent molecular weight of DNase II was ~28 kDa, which is smaller than the full-length DNase II. All the DNase II in BM-cDCs seems to be processed by cathepsin L [23] . No alteration in DNase II expression was found in Tlr9 −/− or Ifnar1 −/− BM-cDCs. Confocal microscopy was next performed. The DNase II mAb stained WT and Ifnar1 −/− , but not Dnase2a −/− Ifnar1 −/− BM-cDCs, with a punctate distribution ( Supplementary Fig. 4b ). When compared with a variety of organelle markers, low but significant co-localization was found with the lysosome marker LAMP-2 and with wheat germ agglutinin (WGA) lectin. No apparent co-localization was found with endoplasmic reticulum marker calnexin or early endosome marker EEA1 ( Fig. 5a ). Although DNase II is considered to be localized in lysosomes, a majority of DNase II was outside the lysosomes. BM-cDCs were stimulated with CpG-A, CpG-B or A3′11, and co-localization of DNase II with LAMP-2 was further studied. Interestingly, CpG-A stimulation upregulated DNase II co-localization with LAMP-2, whereas CpG-B stimulation did not ( Fig. 5b,c ). It is possible that DNase II mRNA is induced by CpG-A, leading to DNase II distribution in lysosomes simply due to the increase in DNase II protein. DNase II mRNA expression, however, was not induced by stimulation with CpG-A, CpG-B or lipid A ( Supplementary Fig. 5a ). DNase II trafficking into lysosomes was induced by CpG-A stimulation, whereas A3′11 failed to induce DNase II trafficking into lysosomes ( Fig. 5d ). Next, localization of CpG-A, CpG-B and A3′11 in lysosomes was examined. Only CpG-A showed co-localization with LAMP2 ( Fig. 5e ). Finally, DNase II was co-stained with CpG-A, CpG-B or A3′11. DNase II co-localization with A3′11 is significantly lower than that with CpG-A or CpG-B ( Supplementary Fig. 5b ). These results suggest that only CpG-A is able to traffic to lysosomes and thereby recruit DNase II into lysosomes. 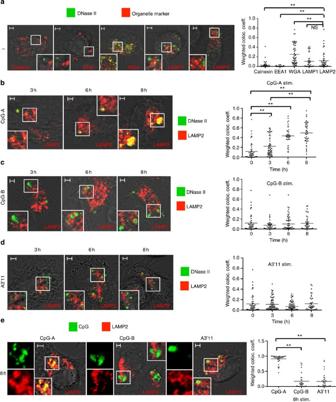Figure 5: DNase II trafficking into lysosomes on CpG-A stimulation in BM-cDCs. (a) Confocal images of BM-cDCs showing DNase II (green) together with organelle markers (red) for endoplasmic reticulum (calnexin), early endosomes (EEA-1), WGA lectin and lysosomes (LAMP-1 and LAMP-2). Confocal images showing co-localization of DNase II (green) and LAMP-2 (red) after stimulation with CpG-A (b), CpG-B (c) or A3′11 ODN (d). (e) Confocal images showing CpG-A, CpG-B, or A3′11 ODN (green) with LAMP-2 (red). Statistical analyses are also shown on the right, respectively (a–e). Statistical analyses were calculated using the Student’st-test (**P<0.01; ns. not significant). Scale bars, 2 μm (at the corners). Weighted co-localization coefficient was used for analyses. Figure 5: DNase II trafficking into lysosomes on CpG-A stimulation in BM-cDCs. ( a ) Confocal images of BM-cDCs showing DNase II (green) together with organelle markers (red) for endoplasmic reticulum (calnexin), early endosomes (EEA-1), WGA lectin and lysosomes (LAMP-1 and LAMP-2). Confocal images showing co-localization of DNase II (green) and LAMP-2 (red) after stimulation with CpG-A ( b ), CpG-B ( c ) or A3′11 ODN ( d ). ( e ) Confocal images showing CpG-A, CpG-B, or A3′11 ODN (green) with LAMP-2 (red). Statistical analyses are also shown on the right, respectively ( a – e ). Statistical analyses were calculated using the Student’s t -test (** P <0.01; ns. not significant). Scale bars, 2 μm (at the corners). Weighted co-localization coefficient was used for analyses. Full size image TLR9 responses to bacterial DNA require DNase II CpG-A and CpG-B are artificially modified by phosphorothioated backbone, which is not seen in naturally occurring DNA. To ask the role of DNase II in TLR9 responses to a longer DNA fragment, a randomly chosen complementary DNA fragment of 0.74 kb was amplified by PCR and used to stimulate TLR9. WT, Tlr9 −/− and Tmem173 −/− BM-cDCs were stimulated with the 0.74-kb dsDNA fragment complexed with or without LF. IL-12p40 production was induced in WT but not in Tlr9 −/− or Tmem173 −/− BM-cDCs ( Fig. 6a ), demonstrating that IL-12 p40 production induced by the 0.74-kb dsDNA fragment is dependent on TLR9. Although BM-cDCs expressed STING mRNA ( Supplementary Fig. 6 ) and responded to a STING ligand 3′3′ cGAMP ( Supplementary Fig. 1b,c ), they failed to produce IL-12p40 when stimulated with dsDNAs, which were known to activate STING ( Supplementary Fig. 1b,c ). Whereas STING induces type I IFN production in dsDNA-stimulated DCs [24] , STING also induces DCs to suppress Th1 responses [24] . Considering that IL-12 is a Th1 cytokine, it might be reasonable that the STING pathway poorly induced IL-12p40 in BM-cDCs. 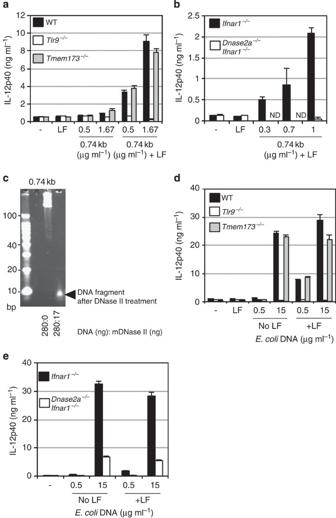Figure 6: DNase II is required for TLR9 response to long DNA fragment and bacterial DNA. (a,d) WT,Tlr9−/−andTmem173−/−BM-cDCs were stimulated with 0.74 kb DNA fragment (a) orE. coliDNA (d) with or without LF. IL-12p40 production was measured by ELISA assay. The results are represented by the average values with s.d. from triplicates. (b,e)Ifnar1−/−orDnase2a−/−Ifnar1−/−BM-cDCs were stimulated with 0.74 kb DNA fragment (b) orE.coliDNA (e) complexed with LF or not. (c) TBE gel electrophoresis of 0.74 kb DNA fragment left untreated or incubated with WT DNase II for 24 h. The arrowhead indicates the cleaved fragments remained after DNase II treatment. Figure 6: DNase II is required for TLR9 response to long DNA fragment and bacterial DNA. ( a , d ) WT, Tlr9 −/− and Tmem173 −/− BM-cDCs were stimulated with 0.74 kb DNA fragment ( a ) or E. coli DNA ( d ) with or without LF. IL-12p40 production was measured by ELISA assay. The results are represented by the average values with s.d. from triplicates. ( b , e ) Ifnar1 −/− or Dnase2a −/− Ifnar1 −/− BM-cDCs were stimulated with 0.74 kb DNA fragment ( b ) or E.coli DNA ( e ) complexed with LF or not. ( c ) TBE gel electrophoresis of 0.74 kb DNA fragment left untreated or incubated with WT DNase II for 24 h. The arrowhead indicates the cleaved fragments remained after DNase II treatment. Full size image Next, Ifnar1 −/− and Dnase2a −/− Ifnar1 −/− BM-cDCs were stimulated with the 0.74 kb DNA/LF complex. IL-12p40 production was detected in Ifnar1 −/− but not in Dnase2a −/− Ifnar1 −/− BM-cDCs ( Fig. 6b ). These results demonstrate a role of DNase II in TLR9 responses to long dsDNA fragment. If DNase II is required, short DNA fragments should be detectable after digestion with DNase II. As expected, about 10-bases DNA fragments were detected after 24 h of DNase II treatment ( Fig. 6c ). To address a role of DNase II in TLR9 responses to bacterial DNA, BM-cDC responses to Escherichia coli DNA was studied. WT, Tlr9 −/− and Tmem173 −/− BM-cDCs were stimulated with E. coli DNA with or without LF. IL-12p40 production was completely dependent on TLR9 even in the presence of LF. As in the case of the 0.74-kb dsDNA fragment, Tmem173 −/− BM-cDCs responded to E. coli DNA as much as WT BM-cDCs ( Fig. 6d ). IL-12p40 production was detected in Ifnar1 −/− but not in Ifnar1 −/− Dnase2a −/− BM-cDCs ( Fig. 6e ). These results demonstrate that DNase II is required for TLR9 activation by bacterial DNA. The present study has shown that DNase II is selectively required for CpG-A, but not CpG-B. CpG-A was cleaved into a half-sized fragment by DNase II and the 3′11-13-mer fragments of CpG-A activated TLR9 in the absence of DNase II. The CpG dinucleotide, which is essential for TLR9 activation, is present in the 3′11-13-mer but not in the 3′ 9-mer. Considering that the 3′10-mer ODN starting with CpG was inactive, an additional ‘T’ is required on the 5′-side of CpG sequence. In this regard, it is of note that the 3′11-mer is similar to CpG-B ODNs in starting with the 6-mer sequence 5′-TCGTCg-3′ ( Fig. 4b ). CpG-A has the CpG dinucleotide in the palindromic, loop-forming region. The CpG motif in the loop is likely to be inactive and CpG-A digestion by DNase II would generate the fragment starting with the 6-mer CpG-containing sequence. As short as 5-mer or 6-mer sequence containing the CpG dinucleotide is able to activate human and mouse DCs [25] , [26] . Considering that A3′11 more strongly bound to mouse TLR9 ectodomain than the full-length CpG-A, the loop structure of CpG-A might inhibit its interaction with TLR9. Both the 0.74-kb DNA fragment and bacterial genomic DNA required DNase II to stimulate TLR9. TLR9 would not be able to directly sense a long dsDNA fragment. DNase II cleaved 0.74 kb DNA to about 10-mer short fragments, which would include a fragment starting with the CpG-containing active sequence such as 5′-TCGTCG-3′. These results suggest that TLR9 is optimized to sense short DNA fragments generated by DNase II-mediated digestion. Recently, RNA:DNA double-stranded hybrids are shown to activate TLR9. However, the ssDNA fragment from RNA:DNA hybrids failed to activate TLR9 (ref. 27 ), probably due to the absence of the CpG motif. RNA:DNA hybrids may be distinct from CpG-containing ssDNA in the way acting on TLR9. DNase II was required for TLR9 responses to bacterial DNA, whereas RNA:DNA hybrids are formed during retroviral infection [27] . It is important to study the role of DNase II in viral infection as well as in bacterial infection. If CpG-A is cleaved into a CpG-B-like fragment for TLR9 activation, it is hard to explain the difference between CpG-A and CpG-B. On CpG-A stimulation, TLR9 induces IFN-α in the LAMP-2 + compartment [22] . CpG-A and DNase II were also detected in such LAMP-2 + compartment. In contrast, CpG-B did not show co-localization with LAMP-2 and CpG-B stimulation did not induce DNase II trafficking to the LAMP-2 + compartment. A3′11, which is similar to CpG-A fragment after DNase II digestion, was similar to CpG-B in distributing outside the lysosomes. CpG-A, but not CpG-B, spontaneously forms nanoparticles, which is similar to virus particles [5] . DNase might interact with such CpG-A nanoparticles and traffic together to the LAMP-2 + compartment, where CpG-A cleavage occurs and TLR9 is activated by the cleaved fragments generated. A previous study showed that in BM-pDCs CpG-A is retained in endosomes where the downstream signalling adaptor MyD88 and transcription factor IFN regulatory factor 7 are recruited [20] . In this previous study, TLR9 distribution in BM-pDCs is not directly shown [20] . In contrast, CpG-A is rapidly transferred to lysosomes in BM-cDCs [20] , which is consistent with the present study. In BM macrophages, CpG-A-stimulated TLR9 traffics to LAMP-2 + lysosomes [22] . pDCs may be distinct in CpG-A trafficking. It is important to study distribution of both TLR9 and CpG-A in all the cell types. It remains to be determined where CpG-A and genomic DNA are cleaved by DNase II and where TLR9 is activated by cleaved fragment in BM-pDCs. DNase II is ubiquitously expressed and its mRNA does not show any drastic change after cell activation ( Supplementary Fig. 5a ). Given that DNase2a −/− mice suffer from spontaneous, systemic lethal inflammation, DNase II has a role in steady-state degradation of DNA in a variety of cells. However, most of the DNase II was detected outside the LAMP-2 + compartment in the resting state and recruited into the LAMP-2 + compartment after CpG-A stimulation, indicating that DNA digestion by DNase II can be upregulated by recruitment of DNase II into the lysosomes, where DNase activity is maximized. It is interesting to study DNase II recruitment during viral infection or tissue damages. In the absence of DNase II, the STING pathway is constitutively activated [15] , whereas TLR9 activation was found to be impaired as found in this study. Engulfed apoptotic DNA in the lysosomes is likely to leak into the cytoplasm and activate the STING pathway. In contrast to TLR9, cytoplasmic DNA sensors may be able to sense uncleaved, long DNA fragments. DNase II seems to positively regulate endosomal DNA sensing and negatively regulate cytoplasmic DNA-sensing. In conclusion, the present study demonstrates a key role of DNase II in DNA sensing by TLR9. Mice WT C57BL/6 mice were purchased from Japan SLC. All the mutant mice were backcrossed to the C57BL/6 strain as indicated below. The Tlr9 −/− mice ( N >8) were a gift from Professor Shizuo Akira (Osaka University, Osaka, Japan). The Ifnar1 −/− mice ( N >6) were purchased from B&K Universal, while the Dnase2a +/− mice ( N >7) were purchased from RIKEN BioResource Center. The Dnase2a −/− Ifnar1 −/− mice were generated by crossing the Ifnar1 −/− and Dnase2a +/− mice. The DNase II conditional knockout mice ( Dnase2a flox/+ ) ( N >7) was also purchased from RIKEN BioResource Center [12] . The Dnase2a flox/flox Tie2 Cre mice were generated by mating the Dnase2a flox/+ and Tie2-Cre transgenic mice ( N >13) (Jackson Laboratory). The Tmem173 −/− mice were generated by Professor Glen N. Barber (University of Miami, Florida, USA) ( N >12). For experiments, 6- to 8-week-old age-matched male mice were used. The animals were kept in a specific pathogen-free environment within the animal facility in the Institute of Medical Science, the University of Tokyo. All animal experiments were approved by the Animal Care and Use Committee, strictly performed in accordance to the institutional ethical guidelines issued by the University of Tokyo. Induction of bone marrow-derived cells BM-cDCs were induced with 10 ng ml −1 of murine granulocyte-macrophage colony-stimulating factor (Peprotech) for 7 days in complete RPMI medium (10% fetal bovine serum, penicillin/streptomycin/l-glutamine, 50 μM 2-ME). For BM-pDCs, BM cells were cultured with 100 ng ml −1 of fms -like tyrosine kinase-3 ligand (Flt3L, Peprotech) for 7 days and CD11c + B220 + cells were sorted before analysis. Ligands Full-sized CpG-A (2,216, sequence 5′- ggGGGACGATCGTCgggggg -3′), all the listed short CpG-A sequences in Fig. 4b , RNA9.2s-DR and the biotinylated A3′11 ODN or CpG-A were synthesized by Hokkaido System Science. CpG-B (1,668, sequence 5′- tccatgacgttcctgatgct -3′) was synthesized by FASMAC. Nucleotides in upper case represent phosphodiester linkage, whereas those in lower cases were phosphorothioate modified. The endotoxin-free double-stranded genomic E. coli DNA, Poly(I:C), 3′3′ cGAMP, ISD, poly(dA:dT) and 5′ppp-dsRNA were purchased from Invivogen. DNA of 741 bp in length was generated by PCR reactions. The sequence was based on the transcript for 14-3-3γ (321-1060). The PCR products were purified with the Wizard SV GEL and PCR Cleanup system (Promega) and eluted with milliQ H 2 O. For treatments with PCR product, DNA was pre-incubated with Lipofectamine 2000 Reagent (Invitrogen) at room temperature for 20 min, following the manufacturer’s instructions before addition. Purification of mouse DNase II proteins The murine WT or mutant Dnase2a (with flag tag) was expressed in Ba/F3 cells. Culture supernatant from these cells was collected and purified with flag peptide (MBL International). For quantification, each of the purified proteins was run in a SDS–PAGE and stained with the SilverQuest Silver staining kit (Invitrogen). The band intensities were then measured using Photoshop (Adobe). The silver staining image shown in Fig. 3a have been cropped for presentation. Full-size images are presented in Supplementary Fig. 8 . DNase II activity assay The activity assay was based on previous work, with slight modifications [18] . The WT or mutant purified DNase II protein (10–50 ng) was incubated with 500 ng plasmid DNA in the activity reaction buffer (10 mM Tris/HCl pH 5.3, 5 mM EDTA pH 8.0). The protein/DNA mixture was incubated at 37 °C for 1 h. Immediately after reaction, the mixture was loaded into 1% ethidium bromide-prestained agarose gel for electrophoresis. Preparation of the mouse TLR9 ectodomain The DNA encoding the extracellular domain of mouse TLR9 from aa 26 to 818 with a carboxy-terminal thrombin cleavage site followed by protein A tag were inserted into the expression vector pMT/BiP/V5-His of the Drosophila expression system. Drosophila S2 cells were cotransfected with the TLR9 and pCoHygro vectors. Stably transfected cells were selected in Sf-900 II SFM medium containing 300 μg ml −1 hygromycin. Protein secreted to the supernatant was purified by IgG Sepharose 6 Fast Flow (GE Healthcare) affinity chromatography, followed by Superdex 200 gel filtration chromatography. To mimic the Z-loop processing, the protein was incubated with 1/50 (w/w) V8 protease (Wako) for 12 h to cleave Z-loop and protein A tag. After proteolytic processing by V8 protease, the N- and C-terminal halves of TLR9 remained associated. Z-loop processed TLR9 was further purified by HiTrap SP (GE Healthcare) cation exchange chromatography. Enzyme-linked immunosorbent assay The cytokines IL-12p40, RANTES, IL-6, TNF-α and IFN-α were measured with the ELISA kits from R&D Systems, following the manufacturer’s instructions. Immunoprecipitation Cells were lysed with 1% lubrol lysis buffer (150 mM NaCl, 20 mM Tris/HCl pH 7.4, 1 mM EDTA pH 8.0, 1% lubrol, 10% glycerol and 1 × complete inhibitor from Roche) and immunoprecipitated with the monoclonal antibodies against TLR9 or DNase II conjugated to the N-hydroxysuccinimide (NHS)-activated sepharose 4 fast flow (GE Healthcare). After 2 h, the beads were washed three times and eluted by boiling with sample buffer (0.1 M Tris/HCl pH 6.8, 20% glycerol, 10% SDS, 6% 2-ME, 0.05% bromophenol blue) at 98 °C for 8 min. The samples were subsequently analysed by using SDS–PAGE. For studying the binding of biotinylated CpG DNA with the purified mouse TLR9 ectodomain, Dynabeads MyOne Streptavidin T1 (Life Technologies) was used for immunoprecipitation. The membranes after transfer were either immunoblotted with the home-made anti-TLR9 TIR domain pAb (1:300), the anti-TLR9 N terminus pAb (eBioscience) (1:100), or anti-DNase II pAb (Santa Cruz) (1:400). For the confirmation of endogenous TLR9 expression in BM-cDCs ( Fig. 1b ) and the coimmunoprecipitation of biotinylated CpG with TLR9 ectodomain ( Fig. 4g ), images have been cropped for presentation. Full-size images are presented in Supplementary Figs 7 and 9 , respectively. For immunoprecipitation of the endogenous DNase II using the conjugated monoclonal antibody ( Supplementary Fig. 4a ), the original image has been cropped for presentation. Full-size image is presented in Supplementary Fig. 10 . Flow cytometry For surface CD11b and CD11c staining, BM-cDCs were pre-incubated with anti-CD16/32 antibodies (1:1,000) in FACS buffer (2.5% FCS, 0.02% NaHCO 3 and 0.1% NaN 3 in PBS), to block the Fc receptors. Cells were stained with the following antibodies purchased from eBioscience: CD11b-FITC (M1/70) (1:1,000) and CD11c-PE (N418) (1:1,200). The stained samples were analysed using the BD Biosciences FACSCalibur cytometer and FlowJo software. BM stem cell transduction On Day 1, fluorouracil (Kyowa) was injected intraperitoneally (at 5 mg per mouse) into the mice. On Day 4, empty vector or GFP-tagged DNase II (WT or mutant)-encoding plasmids were transfected into Plat-E cells for retrovirus packaging. Mice were killed on Day 5. BM cells were obtained and maintained in stem cell medium (15% FCS, 10 mM sodium pyruvate, 1 × penicillin–streptomycin–glutamine, 50 μM 2-ME, 10 ng ml −1 murine IL-3, 10 ng ml −1 murine IL-6 and 100 ng ml −1 murine Stem Cell Factor in plain DMEM medium). On Day 7, viral supernatant was collected and transduced into the stem cell with the reagent (10 ng ml −1 murine IL-3, 10 ng ml −1 murine IL-6, 100 ng ml −1 murine Stem Cell Factor and 10 mM sodium pyruvate) added. The transduction procedure was repeated once more on the next day. Ten nanograms per millilitre of murine granulocyte-macrophage colony-stimulating factor was then added to induce differentiation into cDCs. Cells were used on Day 21. The DNase II expression levels after transduction were evaluated with checking the GFP expression by flow cytometry. Murine IL-3, IL-6 and Stem Cell Factor were all purchased from Wako. Generation of the anti-mouse DNase II mAb The mAbs were established by immunizing the Dnase2a −/− Ifnar1 −/− mouse with well-mixed WT DNase II protein-CFA ( v : v =1:1) emulsion intraperitoneally and also injected into the animal’s footpads. The same protein mixture with incomplete Freund's adjuvant (IFA) was used as boost 2 weeks later. Three more boosts were performed by mixing the DNase II protein with PBS. The mouse was killed 1 week after the final boost. Splenocytes were fused with the myeloma cell line SP2/O-Ag, with gentle addition of polyethylene glycol 1,500 (Roche). Fused cells were seeded into 96-well plate and selected with hypoxanthine-aminopterin-thymidine medium after 24 h. Anti-DNase II monoclonal antibody was screened using the Ba/F3 cells stably expressing the WT DNase II on the cell surface via the pDisplay vector (Life Technologies). Hybridoma supernatants were incubated with the above cell line and analysed by flow cytometry. Positive clones were selected and expanded into 24 wells in HT medium. Monoclones were obtained by limiting dilution with young mice thymuses as feeders. CpG-ODN digestion assay CpG-A or CpG-B was incubated with purified murine DNase II protein in sodium acetate reaction buffer (50 mM sodium acetate pH 4.66 plus 5 mM EDTA pH 8.0) for 24 h at 37 °C. Cleaved DNA was analysed by running in 20% Tris/Borate/EDTA (TBE) gel and stained with GelRed nucleic acid stain (Biotum) following the manufacturer’s instructions. Confocal microscopy Cells were seeded onto a glass-bottom plate (Greiner Bio-One) overnight and fixed (after treatment for respective samples) on the next day with 4% paraformaldehyde for 20 min at room temperature. After permeabilization with 0.2% saponin, cells were stained with the following antibodies in combinations or separately: calnexin (Abcam) (1:333), EEA1 (Cell Signaling Technology) (1:200), WGA (Life Technology) (1:200), LAMP2-Alexa Fluor 647 (clone M3/84 from BioLegend) (1:50) and DNase II (homemade) (1:200). All staining procedures were performed at room temperature. The secondary antibody used for calnexin/EEA1 and DNase II were goat anti-mouse Alexa Fluor 647 (1:3,000) (shown as red pseudo-colour) and goat anti-mouse Alexa Fluor 488 (Invitrogen) (1:3,000), respectively. CpG-A (2216) and CpG-B (1668) in Fig. 5f were labelled with rhodamine (shown as green pseudo-colour). The images were viewed and analysed using LSM710 Confocal Microscopy (Carl Zeiss) and ZEN 2009 software. For statistical analysis, weighted co-localization coefficient was used. Statistical analyses All the statistical analyses were calculated using the Student’s t -test. Real-time PCR Transcript expression levels were determined using the TaqMan probes for detecting DNase II (Mm00438463_m1), TLR9 (Mm00446193_m1) or tmem173 (Mm01158117_m1), and β-actin (Mm00607939_s1) (Applied Biosystems). The reactions were run using the StepOnePlus Real Time PCR System (Applied Biosystems). How to cite this article : Chan, M. P. et al . DNase II-dependent DNA digestion is required for DNA sensing by TLR9. Nat. Commun. 6:5853 doi: 10.1038/ncomms6853 (2015).